Complete determination of molecular orbitals by measurement of phase symmetry and electron density Several experimental methods allow measuring the spatial probability density of electrons in atoms, molecules and solids, that is, the absolute square of the respective single-particle wave function. But it is an intrinsic problem of the measurement process that the information about the phase is generally lost during the experiment. The symmetry of this phase, however, is a crucial parameter for the knowledge of the full orbital information in real space. Here, we report on a key experiment that demonstrates that the phase symmetry can be derived from a strictly experimental approach from the circular dichroism in the angular distribution of photoelectrons. In combination with the electron density derived from the same experiment, the full quantum mechanical wave function can thus be determined experimentally. The description of nature on the atomic scale is successfully performed by quantum mechanics, which treats particles as complex wave functions consisting of an amplitude and a phase. Due to the nature of the measurement process, information about the latter is usually lost and only intensities, that is, the absolute square of the wave function, are accessible in an experiment [2] . However, since the phase is the crucial parameter for remarkable effects from chemical bonding to superconductivity its direct measurement is highly desired. Very few experiments provide information about the phase [3] , [4] , [5] , [6] but these do not allow a simultaneous determination of the spatial distribution. In recent years several experimental techniques were used to measure orbital dependent electron densities [7] , [8] , [9] , [10] . Recovering the phase however is if at all only possible by numerical routines [11] , which all require additional assumptions, for example, on the spatial extent of the wave function [12] , and thus intrinsically restrict the significance of the resulting information. In the following, we show that simultaneously accessing the phase symmetry and the intensity is possible by measuring the excitation distributions of electronic states in reciprocal space using angle-resolved photoelectron spectroscopy (ARPES) [9] , [13] , [14] , [15] with circular polarized light [16] , [17] , [18] . On the example of a molecular model system, we show that the resulting interference pattern of different final states is directly connected to the sign symmetry of the phase. This permits the experimental reconstruction of the complete wave function in reciprocal space without guessing important symmetry parameters. The complete real space wave function is then obtained by a subsequent Fourier transformation. Directly recovering the full information of a quantum mechanical system experimentally constitutes a milestone on the way to a comprehensive understanding of nature on the atomic scale. 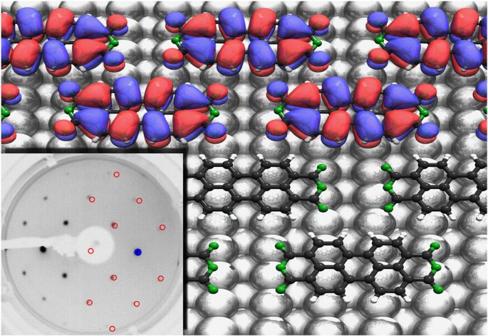Figure 1: Graphical visualization of the investigated monolayer of PTCDA molecules on a Ag(110) surface. The molecules are arranged in the so-called brick wall monolayer in which all the molecules are aligned parallel to the substrate’s [100]-direction. The molecular structure is sketched in the lower part (carbon black, oxygen green, hydrogen white), while in the upper part iso-surface representations of the HOMO are superimposed. Blue and red indicate the different signs of the wave function. The inset at the bottom left shows the experimental validation of the surface preparation by low energy electron diffraction at 16 eV beam energy. The experimental diffraction spots of the PTCDA superstructure correspond to the theoretical prediction (red circles), spots of the substrate are indicated by blue circles. ARPES with circular polarized light Figure 1 presents an artist’s view of the model system 3,4,9,10-perylenetetracarboxylic dianhydride (PTCDA) on a Ag(110) surface. Deposition of a single layer of the planar aromatic molecules leads to a self-organized formation of a commensurate brickwall superstructure in which all molecules are identical and aligned with their long axes parallel to the substrate’s [100]-direction [19] , [20] . The characteristic low-energy electron diffraction pattern is depicted on the lower left of Fig. 1 . 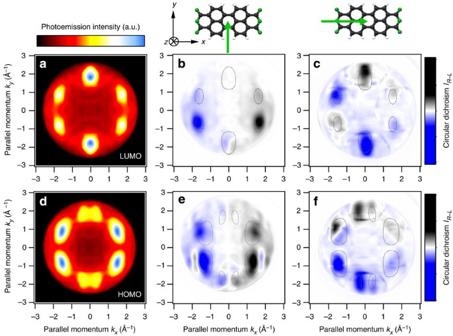Figure 2: CDAD for the PTCDA LUMO and HOMO. (a)k||-dependent photoelectron intensity patterns of the PTCDA monolayer on Ag(110) recorded for the LUMO with a photon energy ofhν=27 eV as the sum of left- and right-handed polarized light, that is, equivalent to unpolarized light. (b) difference between thek||-dependent intensity patterns recorded with right- and left-circular polarized light, that is, the circular dichroismI(kx,ky)R−L, for light incidence along theydirection and (c) for light incidence along thexdirection. For both plots, dotted iso-intensity contours ofaindicate the momentum positions of the molecular structures. (d–f) analogous data for the PTCDA HOMO. On top, the PTCDA molecule is sketched together with green arrows indicating the direction of the incoming light corresponding to the panels below. Figure 2a presents the parallel momentum dependent ( k || =( k x , k x )) photoelectron intensity distributions I ( k x , k y ) recorded at the binding energy of E B =0.8 eV for the lowest unoccupied orbital (LUMO), that is filled due to charge transfer from the substrate and can thus be probed by ARPES [15] , [21] , [22] . The image is the sum of two datasets with left- and right-handed polarized light at 27 eV photon energy, and thus equivalent to unpolarized light. Analogously, Fig. 2d shows the measurement for the highest occupied molecular orbital (HOMO) at the binding energy of E B =2.0 eV. Assuming a plane wave final state for the outgoing photoelectron, the characteristic k || -space intensity patterns can be immediately connected to the absolute square of the Fourier transform of the initial molecular orbital along a spherical cut in k -space, that is, (refs 8 , 14 , 21 ). Figure 1: Graphical visualization of the investigated monolayer of PTCDA molecules on a Ag(110) surface. The molecules are arranged in the so-called brick wall monolayer in which all the molecules are aligned parallel to the substrate’s [100]-direction. The molecular structure is sketched in the lower part (carbon black, oxygen green, hydrogen white), while in the upper part iso-surface representations of the HOMO are superimposed. Blue and red indicate the different signs of the wave function. The inset at the bottom left shows the experimental validation of the surface preparation by low energy electron diffraction at 16 eV beam energy. The experimental diffraction spots of the PTCDA superstructure correspond to the theoretical prediction (red circles), spots of the substrate are indicated by blue circles. Full size image Figure 2: CDAD for the PTCDA LUMO and HOMO. ( a ) k || -dependent photoelectron intensity patterns of the PTCDA monolayer on Ag(110) recorded for the LUMO with a photon energy of hν =27 eV as the sum of left- and right-handed polarized light, that is, equivalent to unpolarized light. ( b ) difference between the k || -dependent intensity patterns recorded with right- and left-circular polarized light, that is, the circular dichroism I ( k x , k y ) R − L , for light incidence along the y direction and ( c ) for light incidence along the x direction. For both plots, dotted iso-intensity contours of a indicate the momentum positions of the molecular structures. ( d – f ) analogous data for the PTCDA HOMO. On top, the PTCDA molecule is sketched together with green arrows indicating the direction of the incoming light corresponding to the panels below. Full size image Recovering the initial orbital in real space from the measured k || -distribution by inverse Fourier transformation requires the phase information, which is not contained in the intensity patterns of Fig. 2a,d . This problem can be overcome by the fact that under certain conditions, deviations from the pure plane wave final state occur. Within the conventional approach presented in ref. 8 , 22 using linearly polarized light, an expansion in partial waves would be similar to the plane wave scenario. By the use of circular polarized light interference effects of the different partial waves of the final state occur [16] , [17] , which are related to the phase distribution within the respective orbital [18] . This is demonstrated by Fig. 2b , which shows the circular dichroism in the angular distribution (CDAD) [17] , [24] , [25] of the LUMO, that is, the difference of the ARPES intensity patterns recorded with right and left circular polarized light I ( k x , k y ) R−L . The existence of the CDAD effect is obvious from the distribution of positive (black) and negative (blue) intensities, which follow the characteristic pattern of the LUMO in Fig. 2a , marked in Fig. 2b by a dotted iso-intensity contour line. Considering the interference of the s- and d-final state channels, the CDAD can in general be calculated analytically and provides the phase of the initial orbital. However, so far, respective calculations have only been performed for atomic p z -orbitals, while for large molecules like PTCDA an exact theoretical description is complicated [17] . As we will demonstrate, the phase symmetry, which allows the reconstruction of the orbital in real space, can be derived from the CDAD if the symmetry of the molecule is known. Reconstruction of the phase symmetry For this purpose, we performed CDAD experiments for different photon incidence directions. While the data in Fig. 2b was derived with light incidence in the plane of the short molecular axis (that is, the y direction according to the coordinate system defined in Fig. 2 ) and the sample normal (that is, z direction), Fig. 2c was recorded with incidence in the x − z plane. For experimental reasons, the incidence perfectly along the y - or the x direction is not possible. In each case, the angle of incidence is 65° against the surface normal, resulting in a projection of the z ′± iy ′ components on the molecular plane (for details of the measurement geometry see supplementary materials ). The PTCDA molecule has C 2 ε symmetry, that is, the individual orbitals are characterized by a twofold rotational symmetry and two mirror planes normal to the molecular plane [26] , [27] . The four different basis functions for the initial state A 1 , A 2 , B 1 , B 2 of the C 2 ε symmetry group show characteristic dichroism signals, because their handedness is different. This becomes obvious when comparing the data in Fig. 2b,c for the LUMO. The CDAD pattern changes clearly when changing the direction of the incoming light. In Fig. 2b , a simple left–right asymmetry is obvious. The decrease of the CDAD signal from the bottom to the top is a consequence of the experimental geometry (for details see Supplementary Fig. 1 and Supplementary Note 1 ). In addition, the CDAD vanishes if the emitted photoelectrons are coplanar with the incident photon beam [17] , [24] , [25] . If the light incidence is within the x − z plane ( Fig. 2c ), the two CDAD maxima on the k x =0 line reverse the sign, that is, in the chosen colour scale the signal on top is black (positive), on bottom blue (negative). The two features at k x =1.7 Å −1 show the same (that is, top black, bottom blue). The signals at k x =−1.7 Å −1 , however, behave differently. Here, the intensity on top is blue, while the one on bottom is black. The CDAD data of the PTCDA HOMO in Fig. 2e,f can be analysed analogously. For both incidence directions, the CDAD of the HOMO displays a different characteristic symmetry pattern: a reversal of the CDAD signs between left and right in Fig. 2e and a reversal between top and bottom in Fig. 2f . Since photon energy-dependent measurements confirm that the final state for the HOMO is the same as for the LUMO (see Supplementary Figs 2 and 3 and Supplementary Note 2 ) and furthermore possible scattering processes can be assumed to be identical [24] , we can conclude that a different symmetry of the initial HOMO and LUMO orbitals leads to the different CDAD results. The fact that the symmetry of the HOMO CDAD is identical for both photon incidence directions shows that the HOMO belongs to the A 1 or A 2 symmetry. Moreover, for a non-vanishing inversion symmetry for both directions only A 2 symmetry is possible. For the LUMO, the symmetry has to be of the type B 1 or B 2 , that is, two different mirror planes must exist. For B 1 symmetry, a nodal plane in the CDAD signal along k x =0 should occur, which is clearly absent in Fig. 2c . Consequently, we can attribute the symmetry B 2 to the LUMO. With the knowledge of the different symmetry representations, the phase symmetry associated with the LUMO and HOMO k || -intensity patterns in Fig. 2a,d can be reasoned. For the HOMO, only an alternating distribution of the sign of the phase fulfils the requirement of full antisymmetry of the A 2 representation. The resulting intensity pattern with superimposed phase is displayed in Fig. 3b . For this reconstruction, we transferred the results of the CDAD—exhibiting the the strongest asymmetry at 27 eV photon energy—to the intensity measurements recorded with 55 eV, because of the larger k || -space available at this higher photon energy. For the LUMO, the B 2 symmetry representation demands for an alternating phase between the two main intensity maxima at k x =0, as well as between the top and bottom signals at k x =±1.7 Å −1 . Consequently, there are two possibilities for the relation of the sign between the k x =0 and the k x =±1.7 Å −1 signals: all signals in the upper part may have the identical or alternating signs. A comparison to theory (see Fig. 3e ) identifies the first option as the correct one. Note that an exact calculation of the photocurrent involving the interference of all photoemission channels is a matter of present research to allow an unambiguous determination of the phase for general systems in near future. The resulting phase distribution for the LUMO is shown in Fig. 3a , with opposite signs for top and bottom and same signs for left and right. 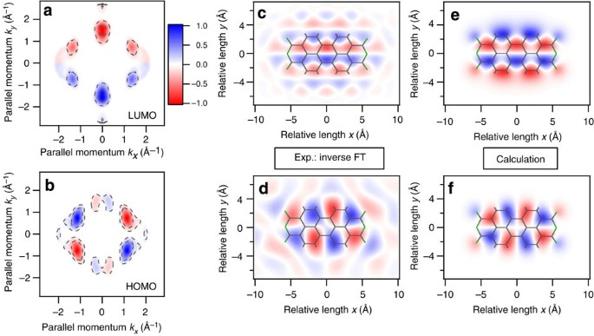Figure 3: Reconstruction of the phase distribution and transformation to real space. k||-dependent photoelectron intensity distributions (hν=55 eV, sum of the left- and right-handed polarized light) of the PTCDA LUMO inaand HOMO inbwith superimposed phase (positive: blue, negative: red) derived from the CDAD. The dashed lines indicate iso-intensity contours of the unpolarized signal. The inverse Fourier transformation leads to the sectional real space views of the real part of the LUMO shown incand the HOMO ind. For illustration, the molecular structure of the PTCDA molecule is superimposed. For comparison, (e) and (f) show the respective real space orbital pictures derived from ab initio calculations for the isolated molecule. Figure 3: Reconstruction of the phase distribution and transformation to real space. k || -dependent photoelectron intensity distributions ( hν =55 eV, sum of the left- and right-handed polarized light) of the PTCDA LUMO in a and HOMO in b with superimposed phase (positive: blue, negative: red) derived from the CDAD. The dashed lines indicate iso-intensity contours of the unpolarized signal. The inverse Fourier transformation leads to the sectional real space views of the real part of the LUMO shown in c and the HOMO in d . For illustration, the molecular structure of the PTCDA molecule is superimposed. For comparison, ( e ) and ( f ) show the respective real space orbital pictures derived from ab initio calculations for the isolated molecule. Full size image Recovering molecular orbitals in real space With this information about the phase distribution, the two-dimensional k -space orbital maps of Fig. 3a,b can be transferred to real space by an inverse Fourier transformation. The results are the sectional views of the real parts of the LUMO and HOMO wave functions as visualized in the Fig. 3c,d , respectively. If compared with the corresponding real space views derived from density functional theory calculations on the free molecule (using the B3LYP 6-311G(d, p) functional) in Fig. 3e,f the agreement is striking. In contrast to the conventional iso-density representation of the theoretical calculated orbitals shown in Fig. 1 , here we show the intensity distributions of the orbital averaged over the top part of the π -orbital. For both the HOMO and LUMO, some distortions due to the hemispherical cut of the measurement in k -space appear. For the LUMO, additional oscillations of the partial charge density in real space emerge at large distances from the molecule and are related to the finite k || -range, which is experimentally accessible. To keep the additional oscillations as small as possible and to increase the resolution in real space, we use the measurements with 55 eV photon energy for the inverse Fourier transform, which allows us to detect photoelectrons with a maximal parallel momentum of . Our study demonstrates the unique potential of angle resolved photoelectron spectroscopy in combination with circular polarized synchrotron light in fully determining the quantum mechanical wave function in real space. Up to now, there are no other experimental techniques that can provide such information appropriately. On the example of the model system PTCDA/Ag(110), we have shown how the phase symmetry can be revealed by group theory with the only presumption being the knowledge of the molecular symmetry, which is well known from both experiments and theory. This constitutes a substantial advance compared with recently published approaches [12] , since the CDAD of photoelectrons is an additional and independent experimental information that can be utilized for the phase reconstruction. In particular, this can provide a route to overcome the primary limitation of the so-called oversampling method applied, for example, in ref. 11 , which relies on guessing the extent of the wave function which is generally not a straightforward task. The phase information derived from our CDAD approach can in fact provide a reference that allows us to adjust the free parameters of mathematical phase retrieval methods thus not only providing the correct phase symmetry of the photoemission intensity patterns but the complete phase of the respective electronic wave function. Sample preparation The Ag(110) substrate was cleaned by cycles of argon ion bombardment (ion energy 2 kV) and subsequent annealing to 800 K. The cleanliness and lateral order were checked by core-level photoelectron spectroscopy and low-energy electron diffraction. The PTCDA brickwall monolayer was prepared in situ by organic molecular beam deposition from a calibrated home-built Knudsen cell (evaporation temperature 640 K) onto the substrate at room temperature [28] , [29] . The PTCDA brickwall monolayer was identified by its very sharp and characteristic low-energy electron diffraction pattern [29] , [30] . k-PEEM The k || -dependent photoemission measurements were performed at the NanoESCA beamline at the synchrotron radiation facility Elettra (Trieste). Photon energies between 25–55 eV were utilized with left-handed circular (LCP) or right-handed circular (RCP) light polarization. The emitted photoelectrons were analysed with respect to their kinetic energy E kin and parallel momentum k || with the NanoESCA photoelectron emission microscope (PEEM, FOCUS/Omicron Nanotechnology) [28] , [30] , [31] , [32] . For photoelectron momentum mapping, the focal plane of the PEEM can be imaged by an additional transfer lens behind the immersion lens objective. This allows a parallel detection of the complete photoemission hemisphere with a momentum resolution of Δ k || =0.05 Å −1 . The overall energy resolution of photon beam and analyser was about Δ E =300 meV, that is, sufficient to distinguish the different PTCDA signals. We continuously checked our measurements for beam damage. No damage was detected on the typical illumination time scale of the experiments of about 10 min. Data acquisition and processing The k || -dependent photoemission intensity patterns in Figs 2a,d and 3a,b were symmetrized according to the C 2 ε symmetry of the adsorbate-substrate system. This reduces the top-bottom intensity asymmetry generated by the | A · k | 2 polarization factor in the photoemission matrix element. To derive the CDAD patterns, we recorded the data with LCP and RCP with the same instrumental parameters (lens settings, integration time and beam position) on the same sample spot. The CDAD patterns can then be calculated by subtracting LCP from RCP measurements (see Supplementary Fig. 1 ). Fourier transformation The inverse Fourier Transformation was performed using an FFT-algorithm. To match the 2 N criterion of the FFT and reduce the coarse in real space, we used a zero padding resulting in an approximately four times larger k x and k y range than actually measured. The resulting photoemission horizon at hν =55 eV is about 3.6 Å −1 . Within this regime, most of the signal of the molecular orbitals is contained. How to cite this article: Wießner, M. et al . Complete determination of molecular orbitals by measurement of phase symmetry and electron density. Nat. Commun. 5:4156 doi: 10.1038/ncomms5156 (2014).